Direct visualization of reversible dynamics in a Si6cluster embedded in a graphene pore Clusters containing only a handful of atoms have been the subject of extensive theoretical and experimental studies, but their direct imaging has not been possible so far, with information about their structure provided mainly by theory. Here we report a direct atomically-resolved observation of a single Si 6 cluster trapped in a graphene nanopore. Furthermore, though electron-beam-induced irreversible atomic displacements have been reported before, here we report a sequence of images that show a reversible, oscillatory, conformational change: one of the Si atoms jumps back and forth between two different positions. Density-functional calculations show that the embedded cluster is exploring metastable configurations under the influence of the beam, providing direct information on the atomic-scale energy landscape. The capture of a Si cluster in a graphene nanopore suggests the possibility of patterning nanopores and assembling atomic clusters with a potential for applications. Silicon clusters have been the subject of a large number of theoretical and experimental studies due to their importance both in fundamental science and potential applications. The structural identification of silicon clusters has been primarily a theoretical search [1] , [2] , [3] , [4] , as experiments such as vibrational [5] , photoemission [6] , infrared multiple photon dissociation spectroscopy [7] and ion mobility measurements [8] have provided limited and indirect information. Recently, nanopore technology has emerged as a powerful tool for single-molecule detection and DNA sequencing. Using an electric field, DNA molecules in an electrolyte solution have been pushed through a graphene pore. As the molecules translocate they partially block ion flow through the pore, detected as a transient decrease in ionic current. Significant information (diameter, length and size) about DNA molecules was obtained through this translocation technique using graphene pores [9] , [10] , [11] . In this paper, we provide direct, atomically-resolved structure information of a single Si 6 cluster trapped in a graphene nanopore using aberration-corrected scanning transmission electron microscopy (STEM). Contrary to previously reported irreversible beam-induced dynamics [12] , [13] , [14] , [15] , [16] , [17] , [18] , [19] , [20] , [21] , [22] , here we report a beam-induced reversible conformational transformation of the trapped Si 6 cluster in a graphene nanopore. Density-functional calculations of an embedded Si 6 cluster are used to probe its bonding to the host graphene lattice and the energy barriers for the conformational transformation. Though the Si atoms are bonded to C atoms with roughly the same bond lengths, the structure of the embedded cluster is only slightly different from that of the free cluster. 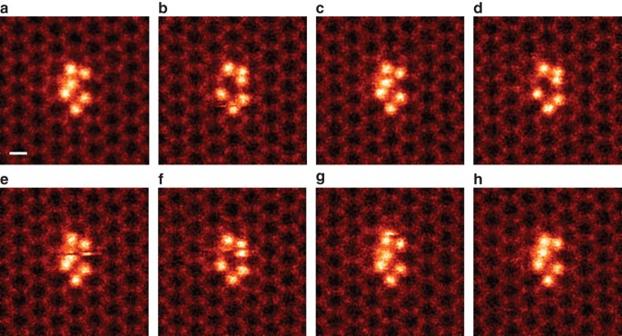Figure 1: Sequential STEM-ADF Z-contrast images of the Si6cluster embedded in a graphene pore (a–h) The images have been low-pass filtered in order to reduce random noise. Scale bar, 0.2 nm. Z-contrast images of a Si 6 cluster trapped in a graphene pore Figure 1 shows a sequential set of annular dark field (ADF) Z-contrast images of a single Si 6 cluster trapped in a graphene nanopore. Electron-beam-induced ejection of carbon atoms and defect creation/migration has been actively studied in graphene and carbon nanotubes [12] , [13] , [14] , [15] , [16] , [17] , [18] , [19] , [20] , [21] , [22] . Contrary to these irreversible dynamics, we find that an oscillatory motion occurs in the trapped Si 6 cluster: one of the Si atoms executes a back-and-forth motion corresponding to the reversible conformational change of the Si 6 cluster in the graphene pore. The acquisition time for the sequential images was ~6 s per frame, which implies that the conformational transformation occurs reversibly in less than ~10 s. Figure 1: Sequential STEM-ADF Z-contrast images of the Si 6 cluster embedded in a graphene pore ( a – h ) The images have been low-pass filtered in order to reduce random noise. Scale bar, 0.2 nm. Full size image Three-dimensional structure characterization The ADF images exhibit two representative stable structures with the oscillating Si atom either at the left or right sites as indicated in Fig. 2a . However, the ADF images do not reveal the full three-dimensional (3D) structure of the cluster. To obtain the pertinent structures, we performed density-functional calculations using the following procedure (see Supplementary Fig. S1 ). (i) The in-plane (xy-plane) atomic positions were extracted from the two fundamental configurations seen in ADF images. (ii) Coordinates in the third-dimension (along the z axis) were assigned to the Si atoms, resulting in nine distinct trial 3D structures for each of the two configurations. (iii) Each trial Si structure was embedded in a graphene pore and in each case the entire system was fully relaxed using first-principles methods. The embedded cluster configuration with the lowest energy corresponding to each of the two fundamental configurations seen in ADF images was then selected (see Supplementary Fig. S2 ). There exists a small deviation in the Si atomic coordinates between the experimental ADF images ( Fig. 2a ) and the calculated structures ( Fig. 2b ). The average Si-C bond length for two clusters is 1.85±0.1 Å, which is similar to that for Si-C bulk (1.89 Å). 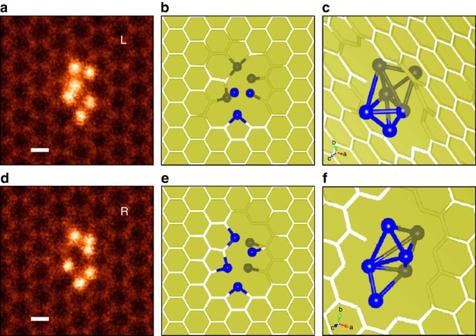Figure 2: 3D structure characterization. (a,d) ADF Z-contrast images of two representative stable Si6cluster configurations embedded in graphene pore. (b,e) The two- and (c,f) 3D structures obtained from first-principles calculations. Si and C atoms below the graphene plane are shaded. L or R labels are used to highlight when the oscillating Si atom is either at the left or right sites. Scale bar, 0.2 nm. Figure 2: 3D structure characterization. ( a , d ) ADF Z-contrast images of two representative stable Si 6 cluster configurations embedded in graphene pore. ( b , e ) The two- and ( c , f ) 3D structures obtained from first-principles calculations. Si and C atoms below the graphene plane are shaded. L or R labels are used to highlight when the oscillating Si atom is either at the left or right sites. Scale bar, 0.2 nm. Full size image Symmetry identification of three Si 6 clusters embedded in graphene pore After some time under the electron beam, one C atom was ejected from the pore edge. Another stable structure configuration was observed. From the ADF Z-contrast image and 3D atomic configuration as shown in Fig. 3a–c , we find that it has a higher-symmetry atomic configuration compared with the previous two clusters. 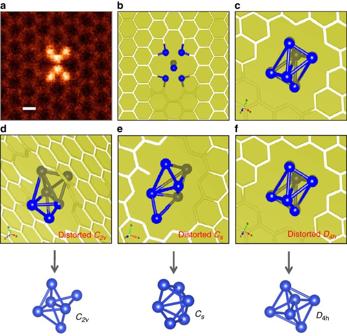Figure 3: Symmetry identification of three Si6clusters embedded in graphene pores. (a) ADF Z-contrast image of the Si6stable cluster embedded in a graphene after the ejection of one C atom. Scale bar, 0.2 nm. (b,c) The two- and 3D structures obtained from first-principles calculations, respectively. Atoms below the graphene plane are shaded. (d–f) The 3D structures of Si6clusters with distortedC2v,CsandD4hsymmetry, respectively. The trapped Si6clusters collapse toC2v,CsandD4hsymmetry configurations when the graphene lattice is removed, as shown in the last row. Figure 3: Symmetry identification of three Si 6 clusters embedded in graphene pores. ( a ) ADF Z-contrast image of the Si 6 stable cluster embedded in a graphene after the ejection of one C atom. Scale bar, 0.2 nm. ( b , c ) The two- and 3D structures obtained from first-principles calculations, respectively. Atoms below the graphene plane are shaded. ( d – f ) The 3D structures of Si 6 clusters with distorted C 2v , C s and D 4h symmetry, respectively. The trapped Si 6 clusters collapse to C 2v , C s and D 4h symmetry configurations when the graphene lattice is removed, as shown in the last row. Full size image To identify the symmetry of the three observed configurations for the Si 6 cluster trapped in the graphene pore, the graphene matrix was removed and the remaining Si 6 were relaxed in free space. We find that the Si 6 clusters collapse to ground-state configurations with full C 2v , C s and D 4h symmetry, respectively, as indicated in Fig. 3d–f . In the free state, the total energy of the Si 6 cluster is essentially the same for the three different configurations with C 2v , C s and D 4h symmetries, and energy barriers between them are small, suggesting a fluxional ground state [4] . However, the present findings show that the clusters trapped in the graphene pore exhibit a distorted version of one of the free-cluster symmetries as the Si atoms are bonded to C atoms at the pore edge. Energy barrier and transition time for conformational transition Through a sequential set of ADF Z-contrast images as shown in Fig. 1 , we have shown that a Si 6 cluster trapped in a graphene pore undergoes reversible conformational transformation. Here we investigate the trajectory and energy barrier for the transformation process using the nudged elastic band method [23] . The initial, three intermediate and the final atomic configurations of the embedded cluster are presented in Fig. 4a–e to show the transformation pathway. The 3D structure of the clusters shows that, though only one Si atom executes an oscillatory motion in the xy-plane, the neighbouring Si and C atoms also move along the z axis in response to the oscillatory motion. 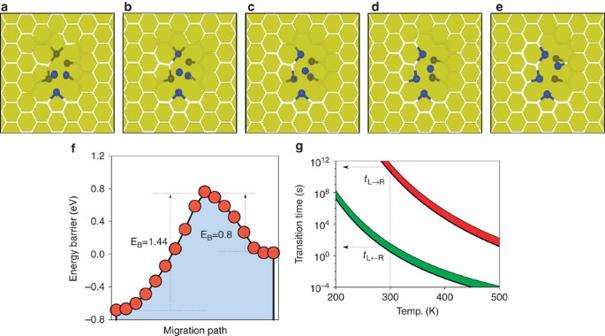Figure 4: Trajectory, energy barrier and transition time for conformational transformation. (a–e) Successive change of the 3D atomic configurations during the conformational transformation. (f) Energy barriers for the conformational transformation. (g) Time required for the transitions from the stable to the metastable Si6clusters (red) and from the metastable to the stable (green) to occur as a function of temperature. The required time for a transition to occur at room temperature is highlighted by the horizontal arrows. Figure 4: Trajectory, energy barrier and transition time for conformational transformation. ( a – e ) Successive change of the 3D atomic configurations during the conformational transformation. ( f ) Energy barriers for the conformational transformation. ( g ) Time required for the transitions from the stable to the metastable Si 6 clusters (red) and from the metastable to the stable (green) to occur as a function of temperature. The required time for a transition to occur at room temperature is highlighted by the horizontal arrows. Full size image We find that the energy barrier ( E B ) for the transformation is 1.44 eV to move out of the ground-state configuration and only 0.8 eV to return to the ground-state configuration as shown in Fig. 4f . According to transition-state theory [24] , the required time for a transformation is given by, where ν is the characteristic attempt frequency of a Si atom (~10 12 –10 13 Hz), k B is the Boltzmann constant and T is the temperature. We estimate that the thermal activation over 1.44 and 0.8 eV energy barriers, at room temperature, takes approximately 10 11 and 10 s, respectively, ( Fig. 4g ). Thus, the observed oscillation of the Si atom in a graphene pore, which takes place in <10 s, is induced by the electron beam. Calculations for scattering cross section and the number of displacements We revealed that the observed conformational transformations are not thermal but rather induced by the beam. However, we still need to understand why the back-and-forth motion of a Si atom corresponding to a reversible conformational transition occurs on a similar time scale (~10 s). To explore this issue, we calculated the scattering cross sections for the two processes. The pertinent theory is described in [25] . The basic point is that during an electron-nucleus scattering event, the energy transfer is given by [25] , where θ is the scattering angle indicated in the inset of Fig. 5 , E is the incident electron energy in MeV and A is the atomic mass number ( A ~28 for Si). For both conformational transitions, the energy transfer E t from the electron beam to the cluster should be greater than the energy barrier E B separating the two minima of the potential energy shown in Fig. 4f . The scattering cross section for an energy transfer E t ≥ E B can be calculated by first determining the minimum scattering angle θ min for which E t = E B using equation (2) ( Fig. 5a ) [25] . 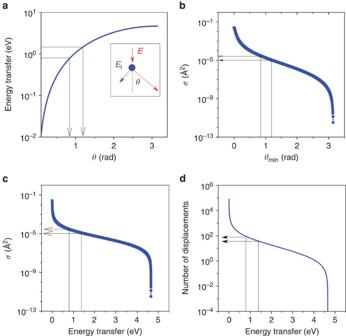Figure 5: Energy transfer, scattering cross section and the number of displacements. (a) Energy transfer in an elastic electron-nucleus collision as a function of the electron scattering angle. Inset: schematic diagram of an elastic scattering event. (b,c) The scattering cross section as a function of the electron scattering angle, energy transfer. (d) The number of displacements of a Si atom as a function of energy transfer. We expect E t ≥ E B for all θ ≥ θ min so that Figure 5: Energy transfer, scattering cross section and the number of displacements. ( a ) Energy transfer in an elastic electron-nucleus collision as a function of the electron scattering angle. Inset: schematic diagram of an elastic scattering event. ( b , c ) The scattering cross section as a function of the electron scattering angle, energy transfer. ( d ) The number of displacements of a Si atom as a function of energy transfer. Full size image in which we use the differential elastic cross section dσ el / dΩ for large-angle scattering and relativistic energies [25] . a H is the Bohr radius (5.29 × 10 −11 m), Z is the atomic number ( Z =14 for Si), E 0 is the electron rest energy, R = a H Z −1/3 and θ 0 = λ/2πR . Based on our energy barrier calculations, in order to move a Si atom from the left site to the right site, E t should be larger than 1.44 eV, for which equation(3) gives σ =1.2 × 10 −5 Å 2 ( Fig. 5b ). For the reverse process, the cross section is 2.8 × 10 −5 Å 2 , only a factor of two larger. Experimentally, we observe a factor of two difference in the forward and reverse rates (see Supplementary Fig. S3 ). As a consequence, the conformational changes induced by electron scattering events occur on the same time scale even though the time scales of the corresponding thermal activations differ by ten orders of magnitude. Figure 5c shows how the scattering cross section depends on the energy transfer E t (from a 60-keV beam electron to a Si atom), which is simply obtained by inserting equation (2) into equation (3). The displacement rate p of an atom [26] is given by the product of the cross section σ and the beam current density j (7.53 × 10 −11 A/Å 2 ). In the STEM experiment, the electron beam scans the specimen from left to the right and from top to bottom staying for 24 μs at each pixel. One Si atom approximately spans 277 pixels. As a result, one can estimate that the electron beam is over a Si atom for about 6.6 ms. By multiplying this dwell time (6.6 × 10 −3 s) by the displacement rate ( p ), we predict 37 displacements of a Si atom from the left site to the right site occurring because of the electron beam. For the reverse process, the number of displacements is expected to be about 87 as indicated in Fig. 5d . Our calculated value is large compared with our experimental observation for the Si atom movement. However, the calculation does not take into account the need for a momentum transfer to be in the direction required to cause a jump, and is therefore expected to be higher than what we observe experimentally. We note, however, that the ratio of observed forward displacements (left to the right) and reverse displacements (right to the left) is indeed about two (see Supplementary Fig. S3 ), which is consistent with the calculated displacement ratio. We further calculated that, under the 60 keV electron beam irradiation, the maximum energy transfer to a Si atom is 4.67 eV, which is lower than the energy for a knock-on displacement of a Si atom out of the cluster, which we calculate to be 6.39 eV. That is why for the most part of the experiment, we observed only reversible conformational transformations instead of ejection of Si atoms from the cluster. We directly observed three stable configurations with different symmetries for Si 6 clusters trapped in a graphene nanopore, and a conformational structural change between two structures induced by energy transferred from the electron-beam in the electron microscope. Specifically, the oscillatory motion of Si atoms between the ground state of the Si 6 cluster and a metastable configuration was directly captured in sequential electron micrographs with atomic resolution. The observations reported here reveal the possibility of identifying the structure and exploring the energy landscape of trapped nanoclusters in graphene pores through electron beam excitation, revealing the metastable atomic configurations that a particular cluster may assume. Density-functional calculations then establish the coordinates in the third dimension (the electron beam direction) from which the energies of each configuration and their transformation pathways can be determined. In this way, our method reveals unique information on the true molecular dynamics of ultrasmall atomic clusters. Though free Si clusters exist in either neutral or charged states, a cluster embedded in a graphene pore cannot exist in a truly charged configuration because of the absence of an energy gap in which a localized state can exist. Nevertheless, we performed calculations to probe the state of an extra electron or hole. In both cases, we find that the extra electron or hole occupies a resonant state at the Fermi energy, but, as expected, there is no charge accumulation at the cluster (see Supplementary Figs S4–S6 ). In summary, the combination of STEM imaging and theoretical calculations has led to the identification of the atomic configuration and dynamics of an ultrasmall cluster embedded in a graphene nanopore. In the present case, the trapping of the cluster occurred during routine chemical vapour deposition growth and/or TEM sample preparation. However, recent experiments have shown that an electron beam can be used to generate pores of particular sizes in graphene [27] . Patterning such graphene pores and subsequently trapping or assembling atomic clusters of specific size or magnetic moment inside them can potentially lead to practical applications. Sample preparation The graphene sample for the study was obtained from Graphene Supermarket. The graphene material was grown on a nickel film on a silicon wafer using a chemical vapour deposition method, and then extracted from the nickel film via chemical etching using concentrated nitric acid, and deposited onto a copper grid. The sample presented single and multi layer graphene regions. The sample then was analysed in the STEM. The trapped Si 6 cluster described in the main text was found in a region of monolayer graphene. STEM-ADF imaging experiments Aberration-corrected STEM-ADF imaging was performed with a Nion Ultra STEM 100, equipped with a cold field emission electron source and a corrector of 3rd and 5th order aberrations [28] . The microscope was operated at 60 kV accelerating voltage, which is below the knock-on radiation damage threshold of graphene. The convergence semi-angle of the incident probe was set to ~30 mrad, and the ADF images were collected from ~54–200 mrad half-angle range. The probe current was set to ~100 pA, containing in a probe of 1.3 Å in diameter. Fast-scan sequential ADF images were acquired from the trapped Si 6 cluster with 24 μs per pixel dwell time, and each frame was recorded with 512 × 512 pixels. The sequential images were then aligned using cross-correlation based on the graphene lattice. All ADF images have been low-pass filtered in order to reduce random noise. Chemical identification of impurity trapped into graphene pore Atom-by-atom chemical analysis was performed based on quantitative intensity analysis of the deconvolved ADF image. The intensity from the impurity atoms is about 3.83 times the intensity obtained from the carbon atoms, which is close to the Z 1.6 ratio of 1:3.87 for Z =6 (C) and Z =14 (Si), respectively [29] . Furthermore, electron energy-loss spectroscopy analysis from a substitutional impurity atom with the same ADF image intensity ratio indicates that the impurities are Si atoms [30] . First-principles calculations First-principles calculations, based on density-functional theory [31] , [32] , were performed using the Vienna Ab initio Simulation Package [33] . The projector-augmented wave method was used to mimic the ionic cores [34] , while the generalized gradient approximation in the Perdew–Burke–Ernzerhof parameterization was employed for the exchange and correlation functional [35] . Atomic positions, as well as lattice parameters were optimized using a conjugate gradient algorithm. Ionic and electronic relaxations were performed by applying a convergence criterion of 5 × 10 −2 eV per Å per ion and 10 −4 eV per electronic step, respectively. A rectangular unit cell of graphene containing 75 C atoms and 6 Si atoms was considered to explore the cluster stabilization in the graphene pore, conformational change and energy barrier. The distance between graphene sheets in neighbouring supercells was set to 14 Å to avoid spurious interactions. A k-point sampling of 4 × 4 × 1 was used for the atomic relaxation. How to cite this article: Lee, J. et al . Direct visualization of reversible dynamics in a Si 6 cluster embedded in a graphene pore. Nat. Commun. 4:1650 doi: 10.1038/ncomms2671 (2013).